MicroRNA-31 negatively regulates peripherally derived regulatory T-cell generation by repressing retinoic acid-inducible protein 3 Peripherally derived regulatory T (pT reg ) cell generation requires T-cell receptor (TCR) signalling and the cytokines TGF-β1 and IL-2. Here we show that TCR signalling induces the microRNA miR-31, which negatively regulates pT reg -cell generation. miR-31 conditional deletion results in enhanced induction of pT reg cells, and decreased severity of experimental autoimmune encephalomyelitis (EAE). Unexpectedly, we identify Gprc5a as a direct target of miR-31. Gprc5a is known as retinoic acid-inducible protein 3, and its deficiency leads to impaired pT reg -cell induction and increased EAE severity. By generating miR-31 and Gprc5a double knockout mice, we show that miR-31 promotes the development of EAE through inhibiting Gprc5a. Thus, our data identify miR-31 and its target Gprc5a as critical regulators for pT reg -cell generation, suggesting a previously unrecognized epigenetic mechanism for dysfunctional T reg cells in autoimmune diseases. T cells serve as a central cellular player in adaptive immunity, and their activation and differentiation are elicited by signals from T-cell receptor (TCR), co-stimulatory receptors and various cytokines [1] . Once activated by an antigen, naive CD4 + T cells proliferate and differentiate into various T helper (T H ) cell subsets, including T H 1, T H 2, T H 17 and regulatory T (T reg ) cells, that release different cytokines and exhibit distinct effector functions [2] . Besides their critical role in driving immune responses against infections, T H 1 and T H 17 cells participate in the pathogenesis of autoimmune inflammatory diseases, such as experimental autoimmune encephalomyelitis (EAE) [3] . Moreover, naive T cells differentiate into T reg cells exhibiting immunosuppressive capacity, and the transcriptional factor FoxP3 controls their development and fucntion [4] , [5] . According to their origins, T reg cells are divided into thymus-derived T reg (tT reg ) cells derived from the thymus, peripherally derived regulatory T (pT reg ) cells generated out of the thymus under various inductive signals, and in vitro -induced regulatory T (iT reg ) cells [6] , [7] . It is now clear that naive CD4 + T cells sorted as FoxP3 − in the thymus possess full potential to differentiate into pT reg cells, thus are potential targets for therapeutic interventions for chronic inflammatory diseases [7] , [8] . Independent on thymus, pT reg cells differentiate in secondary lymphoid organs and tissues, and require TCR signalling and the cytokines TGF-β and IL-2 (ref. 7 ), and only a low antigen dose of a high-affinity TCR ligand is optimal to generate a persistent population of pT reg cells in vivo [9] . So far, dysfunctional T reg cells are identified in several autoimmune disorders including mutiple sclerosis (MS) [10] , [11] , [12] . One of the failures of T reg -cell-mediated immunoregulation is inadequate numbers of T reg cells that may be due to defective induction of pT reg cells in the periphery [13] . Thus, understanding of molecular mechanisms underlying pT reg -cell generation might provide deeper insights into physiological and pathological immune responses in autoimmune inflammatory diseases. MicroRNAs (miRNAs) are single-stranded, small noncoding RNAs located in introns or exons of protein-coding genes as well as in non-coding genes [14] . miRNAs have been implicated in maintaining immune homeostasis during stress, such as inflammation, by regulating gene expression at post-transcriptional level [15] . Several studies have reported that specific miRNA signatures were observed for specialized T-cell subsets, and these miRNAs are dynamically regulated during T-cell maturation [16] , [17] . Dicer and Drosha are two essential components for the generation of miRNA, and loss of these factors leads to defects in lymphocyte differentiation and autoimmune inflammation [18] , [19] . Recently, accumulating evidence has demonstrated that miRNAs are also crucial for T reg -cell development, function and stability [17] , [18] , [19] , [20] . T reg cells display a set of miRNAs that is distinct from conventional T cells [21] . However, intrinsic miRNAs involved in the polarization of T reg cells from naive T cells in vitro and in vivo settings are largely undetermined. In this study, we showed that miR-31 expression was triggered by TCR signalling, and downregulated by TGF-β1-induced FoxP3. The conditional deletion of miR-31 in CD4 + T cells led to enhanced induction of pT reg cells in the periphery, and decreased severity of EAE. Retinoic acid (RA) regulates the expression of genes required for cell proliferation, differentiation and survival by binding its nuclear retinoic acid receptors (RARs) and retinoid X receptors (RXRs) [22] . Although RA has been shown to enforce pT reg -cell generation [23] , the mechanism by which RA promotes pT reg -cell induction is ill-defined. Unexpectedly, we here identified Gprc5a as a direct target of miR-31. Gprc5a is also known as retinoic acid-inducible protein 3 harbouring the functional RAR/RXR binding sites of RA in its core promoter [24] . Gprc5a was targeted by miR-31 through direct binding to its 3′-untranslated regions (3′-UTR), and its deficiency resulted in the impairment of pT reg -cell induction and increased EAE severity. Thus, our findings demonstrated that miR-31 negatively regulated pT reg -cell generation by targeting Gprc5a, suggesting a novel epigenetic mechanism for impaired pT reg -cell induction in autoimmunity. miR-31 expression is triggered by TCR signalling Report of FoxP3 mRNA harbouring the target sequence of miR-31 promoted us to investigate its role in the induction and/or function of T reg cells which are vital for preventing autoimmune disease [21] . We induced EAE, an animal model of MS, with myelin oligodendrocyte glycoprotein peptide (MOG 35–55 ) in mice to investigate expression pattern of miR-31 in pathogenic T cells in the tissue-specific autoimmune inflammation. miR-31 expression was assessed in splenocytes and sorted CD4 + T cells at day 10 post immunization. We found that the expression of miR-31 was significantly increased in both splenocytes and pathogenic CD4 + T cells in EAE mice compared with healthy controls ( Fig. 1a ). We next stimulated the TCR of naive T (CD4 + CD25 − CD62L high ) cells with plate-coated anti-CD3- and soluble anti-CD28-specific antibodies, and we detected that the miR-31 expression was increased ∼ 125-fold in activated CD4 + T cells compared with untreated naive T cells ( Fig. 1b ). Together, these data suggest that TCR signalling induces miR-31 expression in CD4 + T cells. 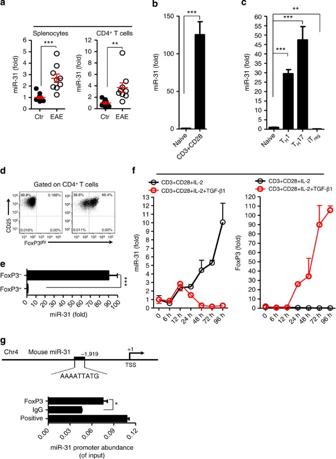Figure 1: TCR signalling triggers expression of miR-31 that is downregulated by TGF-β1-induced FoxP3. (a) qPCR analysis of miR-31 expression in total splenocytes and sorted CD4+T cells from healthy controls (Ctr) or EAE mice (n=9–11) 10 days post immunization. (b) miR-31 expression in naive T cells alone or cultured with anti-CD3, anti-CD28 mAb for 3 days (n=4). (c) qPCR analysis of miR-31 expression in naive T cells and polarized TH1, TH17 and iTregcells (n=4 per group); results are presented relative to miR-31 expression in isolated cells of control mice as inaor in naive T cells as inb,c. (d) Representative flow cytometry of FoxP3gfpexpression in naive T cells cultured with anti-CD3, anti-CD28 mAb and rmIL-2 in the absence (left panel, FoxP3−T cells) or presence (right panel, FoxP3+T cells) of TGF-β1 for 3 days. Numbers adjacent to outlined areas indicate per cent cells in each. (e) qPCR analysis of miR-31 expression in sorted FoxP3−and FoxP3+T cells (n=4 per group). (f) The time course of miR-31 and FoxP3 expression in naive T cells activated by anti-CD3, anti-CD28 mAb and rmIL-2 in the absence or presence of TGF-β1 for 96 h (n=3 per group; results presented as inb). (g) FoxP3 was immunoprecipitated from iTregcells. Immunoprecipitates were assayed for the expression levels ofmiR-31promoter. **P<0.01, ***P<0.001, two-tailed Student’st-test. Data are from one experiment representative of three (a–e) or two (f,g) independent experiments (mean±s.e.m.). Figure 1: TCR signalling triggers expression of miR-31 that is downregulated by TGF-β1-induced FoxP3. ( a ) qPCR analysis of miR-31 expression in total splenocytes and sorted CD4 + T cells from healthy controls (Ctr) or EAE mice ( n =9–11) 10 days post immunization. ( b ) miR-31 expression in naive T cells alone or cultured with anti-CD3, anti-CD28 mAb for 3 days ( n =4). ( c ) qPCR analysis of miR-31 expression in naive T cells and polarized T H 1, T H 17 and iT reg cells ( n =4 per group); results are presented relative to miR-31 expression in isolated cells of control mice as in a or in naive T cells as in b , c . ( d ) Representative flow cytometry of FoxP3 gfp expression in naive T cells cultured with anti-CD3, anti-CD28 mAb and rmIL-2 in the absence (left panel, FoxP3 − T cells) or presence (right panel, FoxP3 + T cells) of TGF-β1 for 3 days. Numbers adjacent to outlined areas indicate per cent cells in each. ( e ) qPCR analysis of miR-31 expression in sorted FoxP3 − and FoxP3 + T cells ( n =4 per group). ( f ) The time course of miR-31 and FoxP3 expression in naive T cells activated by anti-CD3, anti-CD28 mAb and rmIL-2 in the absence or presence of TGF-β1 for 96 h ( n =3 per group; results presented as in b ). ( g ) FoxP3 was immunoprecipitated from iT reg cells. Immunoprecipitates were assayed for the expression levels of miR-31 promoter. ** P <0.01, *** P <0.001, two-tailed Student’s t -test. Data are from one experiment representative of three ( a – e ) or two ( f , g ) independent experiments (mean±s.e.m.). Full size image Because the TCR signal coordinating with lineage-specific cytokines triggers naive T cells to differentiate into specialized effector cells, we sought to examine miR-31 expression in different T-cell subsets. We differentiated naive T cells in vitro under polarizing conditions for the generation of T H 1, T H 17 and iT reg cells in cultures as these T-cell subsets are critical in the pathology of EAE [25] , [26] , [27] . At 4 days after activation, miR-31 expression was 29.5-fold higher in T H 1 cells, 47.4-fold higher in T H 17 cells, but there was 5.6-fold reduction in iT reg cells than that of naive T cells ( Fig. 1c ), which suggested a possible regulatory role for miR-31 in CD4 + T-cell lineage differentiation. Because miR-31 has been implicated to negatively regulate FoxP3 expression in human T reg cells [21] , we sought to investigate whether upregulation of miR-31 coincides with downregulation of FoxP3 during iT reg -cell induction. We polarized naive T cells derived from FoxP3 gfp reporter mice into iT reg cells, and examined miR-31 expression in sorted CD25 + FoxP3 − and CD25 + FoxP3 + cells. The miR-31 expression in CD25 + FoxP3 + cells was ∼ 90-fold lower than that in CD25 + FoxP3 − population ( Fig. 1d,e ). These data demonstrate that miR-31 is preferentially diminished in iT reg cells. Although the expression of miR-31 was slightly increased in tT reg and pT reg cells compared with iT reg cells, its expression in either tT reg or pT reg was not significantly different between control and EAE mice, suggesting that T reg cells maintain baseline miR-31 expression in vivo ( Supplementary Fig. 1a ). To further identify why iT reg cells exhibit diminished levels of miR-31, we activated naive T cells with CD3- and CD28-specific antibodies in the absence or presence of TGF-β1, and measured the time-dependent appearance of miR-31. miR-31 abundance was gradually increased during the stimulation with CD3 and CD28 antibodies in the absence of TGF-β1, however, decreased at 12 h when FoxP3 was induced by adding TGF-β1 ( Fig. 1f ). Moreover, TGF-β1 dose-dependently decreased miR-31 expression in iT reg -cell differentiation ( Supplementary Fig. 1b,c ). Together, these data indicate that miR-31 expression might be downregulated by TGF-β1-induced FoxP3 during iT reg -cell induction in vitro . Database analysis revealed one potential FoxP3-binding site in the promoter element at −1919 upstream from the transcription start site (TSS) of mouse miR-31 ( Fig. 1g upper panel). To establish the possible binding of FoxP3 to the putative binding site in the promoter element of miR-31 , we carried out chromatin immunoprecipitation (ChIP) assays. These assays showed a significant recruitment of FoxP3 to the putative miR-31 promoter ( Fig. 1g lower panel). Thus, our results suggest that FoxP3 possibly binds miR-31 promoter and downregulates its expression during iT reg -cell in vitro differentiation. miR-31 conditional deletion ameliorates autoimmune disease To determine whether miR-31 expressed by pathogenic CD4 + T cells is a functionally relevant regulator for the development of autoimmune inflammation, we used homologous recombination to generate mice with a miR-31 allele flanked by loxP sites (floxed; Fig. 2a upper panel). The germline-transmitted mice were crossed with CD4 Cre transgenic mice to achieve a conditional knockout mouse model with a deleted miR-31 allele in CD4 + T cells ( Fig. 2a lower panel). To verify a specific deletion of miR-31 in CD4 + T cells, we designed primers (P1 and P2) spanning the loxP sites (floxed allele, 1,195 bp; deleted allele, 474 bp) and genotyped mice using DNA of either splenocytes or sorted CD4 + T cells derived from miR-31 fl/fl CD4 Cre (cKO) and miR-31 fl/fl control mice ( Fig. 2a ). We detected both floxed and deleted alleles in splenocytes of cKO mice, while only a floxed allele in splenocytes of miR-31 fl/fl control mice, a deleted allele in CD4 + T cells of cKO mice and a floxed allele in CD4 + T cells of miR-31 fl/fl control mice ( Fig. 2b ). Quantitative real-time PCR (qPCR) analysis confirmed a specific miR-31 ablation in CD4 + T cells in cKO mice ( Fig. 2c ). These mice remained healthy without any detectable immune-mediated pathology at least for 32 weeks. By inducing EAE, we demonstrated that the specific miR-31 ablation in CD4 + T cells significantly decreased its severity accompanied by an evident prevention of weight loss in cKO mice compared with miR-31 fl/fl controls ( Fig. 2d,e ). Moreover, the deletion of miR-31 led to a marked decrease in infiltration of inflammatory cells and demyelination in spinal cord of cKO mice with EAE ( Supplementary Fig. 2a–c ). Thus, using genetic approach, we clearly demonstrated the significant impact of miR-31 expressed by CD4 + T cells on the development of autoimmunity. 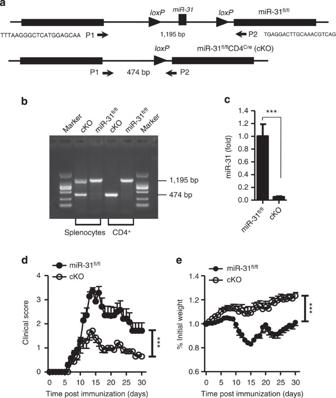Figure 2: Alleviation of autoimmune disease in cKO mice. (a) Schematic representation of themiR-31locus and targeting strategy. Cre-mediated recombination ofloxPsites in mice. Primers (P1 and P2) spanning theloxPsites were designed for genotyping floxed allele (1,195 bp) and deleted allele (474 bp). (b) PCR products of splenocytes and sorted CD4+T cells derived from eithermiR-31fl/flcontrol ormiR-31fl/flCD4Cre(cKO) mice. (c) qPCR analysis to confirm the deletion ofmiR-31in CD4+T cells derived from cKO mice. (d,e) Clinical scores and weight loss (mean±s.e.m.) ofmiR-31fl/flor cKO mice after the induction of EAE were assessed every day (n=7 per group). ***P<0.001, two-tailed Student’st-test forc, one-way analysis of variance fordande. Data are representative of two (c) or three (b,dande) independent experiments (mean±s.e.m.). Figure 2: Alleviation of autoimmune disease in cKO mice. ( a ) Schematic representation of the miR-31 locus and targeting strategy. Cre-mediated recombination of loxP sites in mice. Primers (P1 and P2) spanning the loxP sites were designed for genotyping floxed allele (1,195 bp) and deleted allele (474 bp). ( b ) PCR products of splenocytes and sorted CD4 + T cells derived from either miR-31 fl/fl control or miR-31 fl/fl CD4 Cre (cKO) mice. ( c ) qPCR analysis to confirm the deletion of miR-31 in CD4 + T cells derived from cKO mice. ( d , e ) Clinical scores and weight loss (mean±s.e.m.) of miR-31 fl/fl or cKO mice after the induction of EAE were assessed every day ( n =7 per group). *** P <0.001, two-tailed Student’s t -test for c , one-way analysis of variance for d and e . Data are representative of two ( c ) or three ( b , d and e ) independent experiments (mean±s.e.m.). Full size image miR-31 skews the CD4 T-cell-mediated immune balance To assess how deletion of miR-31 in CD4 + T cells reduced the severity of progressive EAE, we analysed T-cell frequency and activation in non-immunized cKO mice. By flow cytometric analysis, we observed no substantial changes in T-cell numbers and activation status in the thymus in cKO mice compared with miR-31 fl/fl controls ( Supplementary Fig. 3a,b ). T-cell proliferation in response to stimulation via TCR-CD28 was also similar in miR-31 fl/fl and cKO T cells as determined by CellTrace Violet (CTV) fluorescence ( Fig. 3a ). These data suggest that miR-31 is dispensable for T-cell development, activation and proliferation. We next analysed T reg -cell frequency in non-immunized mice, and found that miR-31 deficiency did not change the proportion of T reg cells in the thymus and periphery, indicating that miR-31 had no impact on tT reg and pT reg -cell development ( Supplementary Fig. 4a–c ). T H 1 and T H 17 cells are inflammatory cells that develop during tissue-specific inflammatory responses and play a critical role in enhancing tissue inflammation [25] , [27] . Therefore, we investigated inflamed spleen and central nervous system (CNS) from miR-31 fl/fl and cKO mice for the presence of IFN-γ-producing (T H 1) and IL-17-producing (T H 17) CD4 + T cells during EAE. In contrast to miR-31 fl/fl controls, cKO mice showed a significant reduction of T H 1 and T H 17 cell proportion not only in inflamed spleen ( Fig. 3b,c ) but also in CNS ( Fig. 3d,e ) 14 days post immunization with MOG 35–55 . These data suggest that the development of inflammatory T H 1 and T H 17 cells in cKO mice is impaired during the induction phase of autoimmune disease. We next investigated whether the decreased encephalitogenic potential of CD4 + T cells in cKO mice was a consequence of increased peripheral T reg -cell generation during EAE. On day 14 post immunization, we observed a marked increase in the proportion and absolute numbers of T reg cells in the periphery of cKO mice ( Fig. 3f–h ). Moreover, there was no significant difference of tT reg frequency in miR-31 fl/fl and cKO mice with EAE ( Supplementary Fig. 4d ). Together, these results demonstrate that miR-31 skews the balance between pathogenic T H 1/T H 17 cells and T reg cells in the periphery during autoimmune inflammation. 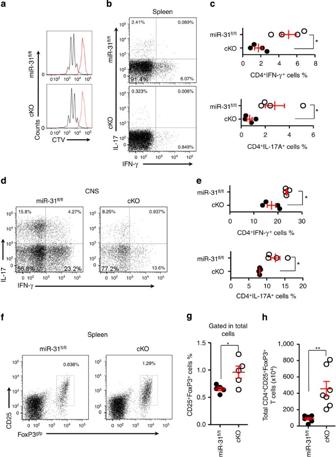Figure 3: miR-31 contributes to altered balance between pathogenic TH1/TH17 cells and Tregcells in autoimmunity. (a) Representative flow cytometric analysis of CTV fluorescence dilution ofmiR-31fl/flor cKO naive T cells cultured with anti-CD3, anti-CD28 mAb and rmIL-2 for 3 days. Red lines indicate non-stimulated controls. (b,c) Flow cytometry of TH1 and TH17 cells in inflamed spleen ofmiR-31fl/fland cKO mice 14 days after the induction of EAE. (d,e) Flow cytometry of TH1 and TH17 cells in CNS ofmiR-31fl/fland cKO mice 14 days after the induction of EAE. (f,g) Flow cytometric analysis of Tregcells in the spleen ofmiR-31fl/fl/FoxP3gfpand cKO/FoxP3gfpmice 14 days after the induction of EAE (n=5, gated on total cells). Numbers in quadrants or adjacent to outlined areas indicate per cent cells in each. (h) Absolute numbers of Tregcells in the spleen ofmiR-31fl/fl/FoxP3gfpand cKO/FoxP3gfpmice 14 days after the induction of EAE (n=7). *P<0.05, **P<0.01, two-tailed Student’st-test. Data are from one experiment representative of at least two independent experiments (mean±s.e.m.). Figure 3: miR-31 contributes to altered balance between pathogenic T H 1/T H 17 cells and T reg cells in autoimmunity. ( a ) Representative flow cytometric analysis of CTV fluorescence dilution of miR-31 fl/fl or cKO naive T cells cultured with anti-CD3, anti-CD28 mAb and rmIL-2 for 3 days. Red lines indicate non-stimulated controls. ( b , c ) Flow cytometry of T H 1 and T H 17 cells in inflamed spleen of miR-31 fl/fl and cKO mice 14 days after the induction of EAE. ( d , e ) Flow cytometry of T H 1 and T H 17 cells in CNS of miR-31 fl/fl and cKO mice 14 days after the induction of EAE. ( f , g ) Flow cytometric analysis of T reg cells in the spleen of miR-31 fl/fl /FoxP3 gfp and cKO/ FoxP3 gfp mice 14 days after the induction of EAE ( n =5, gated on total cells). Numbers in quadrants or adjacent to outlined areas indicate per cent cells in each. ( h ) Absolute numbers of T reg cells in the spleen of miR-31 fl/fl /FoxP3 gfp and cKO/ FoxP3 gfp mice 14 days after the induction of EAE ( n =7). * P <0.05, ** P <0.01, two-tailed Student’s t -test. Data are from one experiment representative of at least two independent experiments (mean±s.e.m.). Full size image miR-31 limits pT reg -cell induction Because miR-31 exhibited a distinct expression pattern in differentiated CD4 + T-cell subsets, we postulated that the intrinsic miR-31 may regulate their in vitro generation. We sorted naive T cells from miR-31 fl/fl and cKO mice, and polarized them into T H 1, T H 17 and iT reg cells under lineage-specific conditions in vitro . After 4 days culture, we found no significant change for the differentiation of T H 1 and T H 17 cells from naive T cells of cKO mice compared with miR-31 fl/fl control mice ( Fig. 4a–d ). Of note, the lack of miR-31 markedly induced iT reg -cell differentiation in culture ( Fig. 4e ). Thus, these data suggest that miR-31 deficiency preferentially enhanced the generation of TGF-β1-induced iT reg cells in vitro . Helios is potentially a marker, which could distinguish tT reg cells from pT reg cells [28] . We injected intravenously bone marrow cells (5 × 10 6 ) from either miR-31 fl/fl or cKO mice into lethally irradiated C57BL/6J recipient mice to generate bone marrow chimeric mice. Eight weeks after bone marrow transplantation, EAE was induced in all chimeric mice. On day 14 post immunization, we analysed the frequency of Helios − FoxP3 + pT reg cells and Helios + FoxP3 + tT reg cells in the spleen of chimeric mice by flow cytometry. By Helios staining, we demonstrated that the conditional deletion of miR-31 led to increased numbers of Helios − pT reg cells, whereas Helios + tT reg cells had no significant change in vivo ( Supplementary Fig. 5 ). Together, our data indicate that miR-31 limits pT reg -cell induction in autoimmunity. We next examined the suppressive capacity of miR-31 fl/fl and cKO T reg cells. CTV dilution determined that cKO T reg cells inhibited T-cell proliferation to the same extent as miR-31 fl/fl T reg cells ( Fig. 4f ). pT reg cells had robust suppression and enhanced stability, suppressed ongoing EAE [29] . Given the fact that pT reg cells converted from conventional T cells play a critical role in the control of development of EAE or other autoimmune diseases [8] , [26] , [30] , [31] , [32] , we here provided strong evidence that promoting generation of pT reg cells by disrupting miR-31 was likely responsible for the observed phenotype. 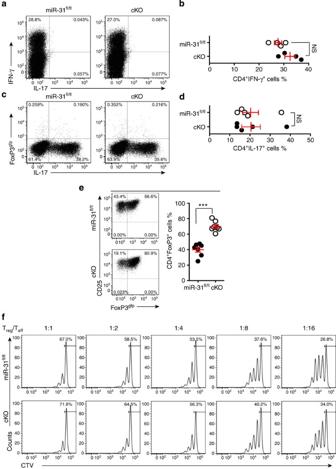Figure 4: miR-31 restrains iTregcell differentiationin vitro. FoxP3gfpreporter mice were crossed with eithermiR-31fl/flor cKO mice. (a–d) Flow cytometry of TH1 and TH17 cells polarized from naive T cells ofmiR-31fl/fl/FoxP3gfpand cKO/FoxP3gfpmice (n=4–5). Numbers in quadrants indicate per cent cells in each. (e) Flow cytometric analysis ofin vitro-induced iTregcells from naive T cells ofmiR-31fl/fl/FoxP3gfpand cKO/FoxP3gfpmice (n=7). Numbers adjacent to outlined areas indicate per cent cells in each. (f) FoxP3gfp+Tregand naive T cells (Teff) were sorted by flow cytometry. The CTV-labelled T cells (1 × 105) were cultured in 96-well plates for 72 h together with a decreasing ratio of sortedmiR-31fl/flor cKO Tregcells in the presence of anti-CD3 (1 μg ml−1) plus γ-irradiated antigen-presenting cells (1 × 105). The suppressive function of Tregcells was determined by the proliferation of activated Teffcells on the basis of CTV dilution. NS, not significant, ***P<0.001, two-tailed Student’st-test. Data are from one experiment representative of at least two independent experiments (mean±s.e.m.). Figure 4: miR-31 restrains iT reg cell differentiation in vitro. FoxP3 gfp reporter mice were crossed with either miR-31 fl/fl or cKO mice. ( a – d ) Flow cytometry of T H 1 and T H 17 cells polarized from naive T cells of miR-31 fl/fl /FoxP3 gfp and cKO/ FoxP3 gfp mice ( n =4–5). Numbers in quadrants indicate per cent cells in each. ( e ) Flow cytometric analysis of in vitro -induced iT reg cells from naive T cells of miR-31 fl/fl /FoxP3 gfp and cKO/ FoxP3 gfp mice ( n =7). Numbers adjacent to outlined areas indicate per cent cells in each. ( f ) FoxP3 gfp+ T reg and naive T cells (T eff ) were sorted by flow cytometry. The CTV-labelled T cells (1 × 10 5 ) were cultured in 96-well plates for 72 h together with a decreasing ratio of sorted miR-31 fl/fl or cKO T reg cells in the presence of anti-CD3 (1 μg ml −1 ) plus γ-irradiated antigen-presenting cells (1 × 10 5 ). The suppressive function of T reg cells was determined by the proliferation of activated T eff cells on the basis of CTV dilution. NS, not significant, *** P <0.001, two-tailed Student’s t -test. Data are from one experiment representative of at least two independent experiments (mean±s.e.m.). Full size image Gprc5a is a target of miR-31 To elucidate the mechanisms, we combined microarray gene expression analysis and target prediction to look for putative targets of miR-31. Using a combination of these two approaches, we identified seven predicted target genes that were upregulated in polarized iT reg cells derived from cKO mice ( Fig. 5a–c ). To confirm accuracy of the microarray data, we validated these potential target genes by increasing sample numbers. We found one predicted target of miR-31, Gprc5a, was significantly upregulated at mRNA levels, and increased by more than 5.0-fold in cKO iT reg cells compared with miR-31 fl/fl controls ( Supplementary Fig. 6 and Fig. 5d ). In contrast to miR-31 fl/fl iT reg cells, Gprc5a protein level was also increased by 1.96-fold in cKO iT reg cells ( Fig. 5e ). Gprc5a was reported to be regulated directly by RA via its receptors, RARs and RXRs [33] , [34] . These nuclear RA receptors bind to the Gprc5a promoter for its transcriptional activity [24] . We next generated a reporter construct that includes the 3′-UTR of Gprc5a mRNA. In contrast to a control construct lacking the target sequence, miR-31 overexpression led to significantly decreased luciferase activity derived from the construct expressing the target sequence ( Fig. 5f,g ). Thus, our data demonstrate that miR-31 is capable of directly targeting a sequence within the 3′-UTR of Gprc5a mRNA and that Gprc5a is one of the key targets of miR-31 in T reg -cell differentiation. 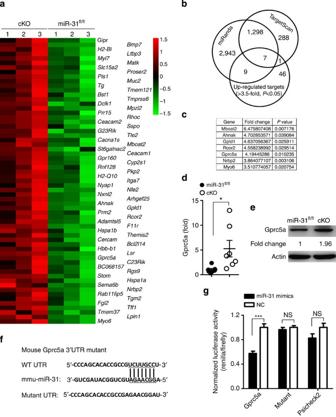Figure 5: Gprc5a is directly targeted by miR-31. (a) Total RNAs of polarized iTregcells derived from 3miR-31fl/flcontrols and 3 cKO mice were used for a microarray analysis (41,174 genes in total). Transcripts of top 63 genes were found to be upregulated in iTregcells of cKO mice. (b,c) TargetScan and miRnada predicted 1,305 potential targets of miR-31. The overlapping seven genes were defined as ACCEPT genes. (d,e) qPCR or western blot analysis of Gprc5a expression in polarized iTregcells derived frommiR-31fl/fland cKO mice. (f) WT and point-mutated 3′-UTR reporter constructs. (g) Luciferase activity was determined in NIH3T3 cells that were transfected with miR-31 mimics and the indicated 3′-UTR reporter construct or with the indicated WT or point-mutated 3′-UTR reporter construct (WT UTR or mutant UTR). Results (d) are presented as the ratio of mRNA to the β-actin, relative to that in controls. *P<0.05; ***P<0.001, NS, not significant, two-tailed Student’st-test. Data (d,eandg) are representative of at least two independent experiments (mean±s.e.m.). Figure 5: Gprc5a is directly targeted by miR-31. ( a ) Total RNAs of polarized iT reg cells derived from 3 miR-31 fl/fl controls and 3 cKO mice were used for a microarray analysis (41,174 genes in total). Transcripts of top 63 genes were found to be upregulated in iT reg cells of cKO mice. ( b , c ) TargetScan and miRnada predicted 1,305 potential targets of miR-31. The overlapping seven genes were defined as ACCEPT genes. ( d , e ) qPCR or western blot analysis of Gprc5a expression in polarized iT reg cells derived from miR-31 fl/fl and cKO mice. ( f ) WT and point-mutated 3′-UTR reporter constructs. ( g ) Luciferase activity was determined in NIH3T3 cells that were transfected with miR-31 mimics and the indicated 3′-UTR reporter construct or with the indicated WT or point-mutated 3′-UTR reporter construct (WT UTR or mutant UTR). Results ( d ) are presented as the ratio of mRNA to the β-actin, relative to that in controls. * P <0.05; *** P <0.001, NS, not significant, two-tailed Student’s t -test. Data ( d , e and g ) are representative of at least two independent experiments (mean±s.e.m.). Full size image Gprc5a is critical for pT reg -cell differentiation Gprc5a was reported to be expressed preferentially in lung tissue and to be a putative lung tumour suppressor gene [35] . The functional analysis of Gprc5a in T-cell differentiation and autoimmunity is not yet performed. We induced EAE, and measured Gprc5a expression in inflamed spleen and sorted CD4 + T cells. In contrast with non-immunized controls, Gprc5a expression was significantly decreased in spleen and CD4 + T cells in EAE mice, and this might be the consequence of increased miR-31 under inflammatory conditions ( Fig. 6a,b ). Western blot analysis confirmed that expression of Gprc5a protein was much lower in spleen and CNS of EAE mice than those of healthy controls ( Fig. 6c,d ). We assessed the role of Gprc5a in pT reg -cell generation using Gprc5a −/− mice [35] . Gprc5a deficiency resulted in a marked decrease in the TGF-β1-mediated induction of iT reg cells, but had no impact on the induction of T H 1 and T H 17 cells ( Fig. 6e and Supplementary Fig. 7a,b ), suggesting that Gprc5a preferentially regulates FoxP3 expression. Thus, our data demonstrate that Gprc5a is a novel regulator in iT reg -cell generation. Interestingly, consistent with the observation in miR-31 cKO mice, we found that Gprc5a deficiency did not affect tT reg -cell generation in healthy mice ( Fig. 6f ). To test the impact of Gprc5a on the T reg -cell response during inflammation, we analysed the frequency of T reg cells in inflamed spleen in Gprc5a −/− mice after the induction of EAE. Gprc5a deficiency resulted in a significant decrease in the percentage of pT reg cells compared with WT controls ( Fig. 6g, h ), suggesting that Gprc5a is critically required for pT reg -cell generation in vivo in autoimmune disease. Notably, Gprc5a −/− mice developed EAE not only much earlier, but also more severe than Gprc5a +/+ mice ( Fig. 6i ). Moreover, an excessive weight loss was displayed in Gprc5a −/− mice compared with Gprc5a +/+ mice ( Fig. 6j ). To further investigate whether miR-31 affects EAE development via regulating Gprc5a in vivo , we generated double knockout (DKO) mice by crossing miR-31 cKO mice with Gprc5a −/− mice. We demonstrated that the severity of EAE was significantly reduced in cKO mice compared with Gprc5a −/− mice, however, the disease phenotype was completely restored when Gprc5a was deleted in the cKO mice ( Supplementary Fig. 7c ). Collectively, our observations indicate that Gprc5a is regulated by miR-31, and functionally involved in the development of EAE. The beneficial effect of RA is possibly due to its stimulation of Gprc5a expression to promote pT reg -cell generation in tissue-specific autoimmune inflammation. 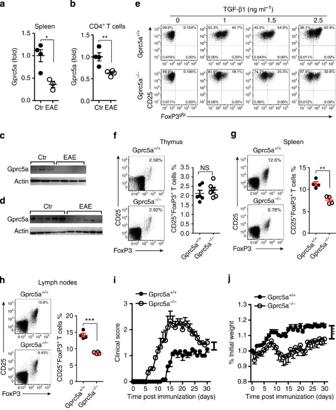Figure 6: Gprc5a deficiency decreases pTreg-cell differentiation and promotes autoimmune inflammation. (a,b) Splenocytes were prepared from unimmunized control mice (Ctr) or EAE mice 10 days after immunization (n=3–4). qPCR analysis of Gprc5a expression in total splenocytes or in sorted CD4+T cells. (c,d) Western blot analysis of Gprc5a in splenocytes and CNS infiltrating cells derived from healthy controls (Ctr) or EAE mice. (e) Naive T cells were sorted fromGprc5a+/+andGprc5a−/−mice. Flow cytometry of polarized iTregcells in the presence of different concentrations of TGF-β1. (f) Flow cytometric analysis of Tregcells in thymus from 6-week-oldGprc5a+/+andGprc5a−/−mice (gated on CD4+T cells). (g,h) Flow cytometric analysis of Tregcells in the inflamed spleen and lymph nodesGprc5a+/+andGprc5a−/−mice 14 days after the induction of EAE (gated on CD4+T cells). Numbers adjacent to outlined areas indicate per cent cells in each. (i,j) Clinical scores and weight loss (mean±s.e.m.) ofGprc5a+/+orGprc5a−/−mice after the induction of EAE were assessed every day (n=7). *P<0.05, **P<0.01, ***P<0.001, NS, not significant, two-tailed Student’st-test fora,b,f,gandh; one-way analysis of variance fori,j. Data are representative of at least two independent experiments (mean±s.e.m.). Figure 6: Gprc5a deficiency decreases pT reg -cell differentiation and promotes autoimmune inflammation. ( a , b ) Splenocytes were prepared from unimmunized control mice (Ctr) or EAE mice 10 days after immunization ( n =3–4). qPCR analysis of Gprc5a expression in total splenocytes or in sorted CD4 + T cells. ( c , d ) Western blot analysis of Gprc5a in splenocytes and CNS infiltrating cells derived from healthy controls (Ctr) or EAE mice. ( e ) Naive T cells were sorted from Gprc5a +/+ and Gprc5a −/− mice. Flow cytometry of polarized iT reg cells in the presence of different concentrations of TGF-β1. ( f ) Flow cytometric analysis of T reg cells in thymus from 6-week-old Gprc5a +/+ and Gprc5a −/− mice (gated on CD4 + T cells). ( g , h ) Flow cytometric analysis of T reg cells in the inflamed spleen and lymph nodes Gprc5a +/+ and Gprc5a −/− mice 14 days after the induction of EAE (gated on CD4 + T cells). Numbers adjacent to outlined areas indicate per cent cells in each. ( i , j ) Clinical scores and weight loss (mean±s.e.m.) of Gprc5a +/+ or Gprc5a −/− mice after the induction of EAE were assessed every day ( n =7). * P <0.05, ** P <0.01, *** P <0.001, NS, not significant, two-tailed Student’s t -test for a , b , f , g and h ; one-way analysis of variance for i , j . Data are representative of at least two independent experiments (mean±s.e.m.). Full size image T reg cells have been reported to be capable of controlling CNS autoimmunity in several CD4 + T-cell-driven EAE models. T reg -cell frequency within the CNS was increased during the recovery phase of actively induced EAE [36] , [37] , and the adoptive transfer of T reg -cells ameliorated EAE symptoms [36] , [38] . Furthermore, depletion of T reg cells with anti-CD25 mAb has been demonstrated to exacerbate EAE [36] . More importantly, reduced T reg -cell proliferative potential and cloning frequency were identified in patients with MS [12] , [39] . Thus, regulators of T reg -cell generation are considered to harbour valuable potential for clinical applications in the treatment of autoimmune disorders. Here, we report that miR-31 expression in CD4 + T cells was triggered by TCR signalling, and downregulated by TGF-β1-mediated FoxP3. Its conditional deletion substantially enhanced the pT reg -cell induction and ameliorated disease severity in the EAE model. Mechanistically, we have proven that by targeting Gprc5a, a known retinoic acid-inducible protein, miR-31 promoted the generation of pT reg cells in vivo . Gprc5a is a functional target of miR-31, and its deficiency resulted in impaired pT reg -cell generation and increased EAE severity. Antigen-specific stimuli delivered through the TCR cooperates with antigen-nonspecific cytokines to support proliferation and differentiation of distinct T H cell subsets [40] . However, it has become increasingly clear that miRNAs, post-transcriptional regulators, are involved in driving T H cell differentiation and lineage commitment [41] . A selective effect of miR-31 on pT reg -cell differentiation could be explained by the differential requirement of TCR signalling in the induction of these T-cell lineages. A low antigen dose of a high-affinity TCR ligand favours to induce pT reg cells in vivo [9] , whereas high doses of TCR stimulation prevents FoxP3 induction and pT reg -cell generation through activating NF-κB signalling [42] . Indeed, we have determined that the activation of NF-κB induced miR-31 expression through a direct binding of p65 to its promoter (to be published elsewhere). Thus, it is possible that in the absence of TGF-β1, TCR stimulation at high doses elicits activation of NF-κB, which directly triggers the expression of miR-31 inhibiting FoxP3 levels in CD4 + T cells. However, TCR stimulation at low doses induces FoxP3, which may downregulate miR-31 expression through binding to its promoter, providing a feedback loop during pT reg -cell differentiation. Several miRNAs have been reported to impact T reg -cell development and function. miR-155 is highly expressed in T reg cells, facilitates T reg -cell homeostasis by repressing Socs1 and its deficiency results in decreased numbers of both tT reg cells and pT reg cells [43] . miR-21 indirectly acts as a positive regulator of human FoxP3 expression [21] . miR-146a is critical for T reg -cell-mediated control of T H 1 responses via targeting Stat1 (ref. 44 ). Despite that miR-17 ∼ 92 is dispensable for the development of tT reg cells in vivo , miR-17 ∼ 92 ablation reduces the frequency of MOG 35–55 -specific pT reg cells during EAE [45] . miR-10a is induced by TGF-β1 and RA, and promotes the differentiation of pT reg cells through inhibiting Bcl-6 (ref. 46 ). Collectively, these T reg -cell-associated miRNAs are all enriched in T reg cells compared with conventional T cells, and function as positive regulators. Our data demonstrated that miR-31 was preferentially diminished in T reg cells, was downregulated by FoxP3, and negatively regulated naive CD4 + T-cell differentiation into pT reg cells. The conditional deletion of miR-31 in CD4 + T cells resulted in enhanced induction of pT reg cells in the periphery, and decreased severity of autoimmune disease. Thus, we highlight miR-31 acts as a negative regulator for pT reg -cell generation in vivo . Although different targets of miR-31 were identified, its similar effect was also reported previously for human T reg cells [21] . Our findings are inconsistent with a recent report which demonstrated that growth factor independent 1 (Gfi-1) was underexpressed in pT reg cells, downregulated by TGF-β1 and limited the pT reg -cell differentiation [47] . miR-31 is the only member of a broadly conserved miRNA ‘seed family’ that is present in vertebrates and Drosophila [48] . miR-31 regulates keratinocyte differentiation through inhibiting hypoxia-inducible factor 1 (ref. 49 ). Furthermore, in contrast to other T-cell subsets, miR-31 has been shown to be downregulated in human T reg cells [21] . This raises the intriguing possibility that miR-31 may be preferentially diminished in T reg cells and its upregulation in CD4 + T cells under inflammatory stress may limit pT reg cell induction in human autoimmune diseases. RA has been proven to facilitate pT reg -cell generation [23] . RA regulates Gprc5a transcriptional activity by binding to its receptors, RARs and RXRs [24] , [33] , [34] . So far, the role of Gprc5a in the T-cell differentiation programme is not investigated. We here showed that Gprc5a deficiency led to a severe defect in in vitro - and in vivo -generation of T reg cells, as well as increased severity of inflammatory CNS phenotypes, indicating that this may be one of the mechanisms by which RA inhibits autoimmune reactions in vivo . However, the molecular mechanism by which Gprc5a promotes T reg -cell generation and suppresses autoimmune disease is subjected to further investigation. Nevertheless, by generating miR-31 and its target Gprc5a DKO mice we clearly show that miR-31 promotes the development of autoimmune disease through inhibiting Gprc5a. In summary, our results demonstrate that miR-31 inhibits pT reg -cell generation through directly targeting Gprc5a, a retinoic acid-inducible protein and promotes autoimmunity, therefore, providing the first in vivo genetic evidence that miR-31 and its novel target Gprc5a are critical intrinsic factors for controlling physiological and pathological immune responses regulated by pT reg cells. Mice C57BL/6J mice (stock number: 000664), B6.Cg- FoxP3 tm2Tch/J mice (stock number: 006772, designated as FoxP3 gfp ) and CD4 Cre mice (stock number: 017336) were purchased from The Jackson Laboratory (Bar Harbor, ME). B6.129S6-Rag2 tm1Fwa N12 ( RAG2 −/− ) mice were purchased from Taconic Labs (Hudson, NY). Gprc5a −/− mice were generated as previously reported [35] . Mice were kept under specific pathogen-free conditions in compliance with the National Institutes of Health Guide for the Care and Use of Laboratory Animals with the approval (SYXK-2003-0026) of the Scientific Investigation Board of Shanghai Jiao Tong University School of Medicine, Shanghai, China. To ameliorate any suffering of mice observed throughout these experimental studies, mice were euthanized by CO 2 inhalation. Generation of miR-31 fl/fl and miR-31 fl/fl CD4 Cre mice The miR-31 locus (mmu-mir31 ENSMUSG00000065408, http://www.ensembl.org/index.html ) is on the chromosome 4 (Mus musculus) and encodes the miR-31 . To create loxP-miR-31-loxP mice, a targeting vector was designed to insert with an frt-flanked PGK-neo cassette and a loxP site upstream of miR-31 , and a second loxP site downstream. LoxP site is a 34 bp length DNA sequence that can be recognized by Cre recombinase catalyses. If two loxP sites are introduced in the same orientation into a genomic locus, expression of Cre results in the deletion of the loxP-flanked DNA sequence. After linearization, the vector was electroporated into 129S6-derived embryonic stem (ES) cells. The collected ES cells were screened with 300 μg ml −1 G418 and 2 μM Gan C for 8 days and ascertained by PCR. The ES cells with right homologous recombination were injected into blastocyst. After birth, the chimeric mice were bred with 129S mice to generate the heterozygotes. At this point, mutant mice were bred with Flp recombinase-expressing mice to remove the frt-flanked neo cassette. The resulting loxP-miR-31-loxP mice were backcrossed into C57BL/6J background for eight generations and bred with CD4 Cre transgenic mice. P1 and P2 were used to genotype the miR-31 floxed allele (1,195 bp) and the miR-31 deleted allele (474 bp). P1, 5′- TTTAAGGGCTCATGGAGCAA -3′; P2, 5′- TGAGGACTTGCAAACGTCAG -3′. Excision by CD4 Cre was complete for all pups used in experiments. In some experiments, these mice were further crossed with FoxP3 gfp mice to generate mice that express green fluorescent protein (GFP) in their T reg cells. Induction of EAE EAE was induced by complete Freund’s adjuvant (CFA)-MOG 35–55 peptide immunization (China Peptides Biotechnology) and scored daily. Briefly, C57BL/6J mice were injected subcutaneously into the base of the tail with a volume of 200 μl containing 300 μg MOG 35–55 peptide emulsified in CFA (Sigma-Aldrich). Mice were also injected intravenously with 200 ng of pertussis toxin (Merck-Calbiochem) on day 0 and 2 post immunization. All the reagents used for in vivo experiments were free of endotoxin. Mice were monitored daily for the development of disease which was scored according to the following scale: 0, no symptoms; 0.5, partially limp tail; 1, completely limp tail; 1.5, impaired righting reflex; 2, hind limb paresis; 2.5, hind-limb paralysis; 3, forelimb weakness; 4, complete paralysis; 5, moribund or death. T-cell isolation and sorting Peripheral T cells were obtained from the spleen and lymph nodes of 6-week-old mice. Naive CD4 + T cells (CD4 + CD25 − CD62L high ) were sorted by FACSAria III (BD Biosciences) after enrichment of CD4 + T cells by the mouse CD4 + T cell Isolation Kit (Miltenyi). For the isolation of naive CD4 + T cells and nT reg cells from Foxp3 gfp mouse, CD4 + CD25 − GFP − CD62L high cells and CD4 + CD25 + GFP + cells were isolated, respectively. Cell purity was >94% as determined by flow cytometry. CNS-infiltrating mononuclear cells from EAE mice were prepared by Percoll (GE Healthcare) gradient separation. In vitro T reg -cell differentiation All the cultures of T cells used RPMI-1640 medium (Gibco) supplemented with 10% heat-inactivated fetal bovine serum (Gibco), 2 mM L-glutamine (Gibco), 100 IU ml −1 penicillin, 100 μg ml −1 streptomycin, 10 mM HEPES (Gibco) and 5 mM β-mercaptoethanol (Gibco). The naive CD4 + CD25 − Foxp3 gfp- CD62L hi T cells were activated with plate-bound anti-CD3 (5 μg ml −1 ; 145-2C11; BD Biosciences) plus soluble anti-CD28 (2 μg ml −1 ; 37.51; BD Biosciences). T H 1-cell differentiation conditions included 10 ng ml −1 rmIL-12 (R&D Systems) and 10 μg ml −1 anti-IL-4 (11B11; Biolegend). The T H 17 cell differentiation conditions included 20 ng ml −1 rmIL-6 (R&D Systems), 3 ng ml −1 rmTGF-β1 (R&D Systems), 10 μg ml −1 anti-IL-4 (11B11; Biolegend) and 10 μg ml −1 anti-IFN-γ (XMG1.2; eBioscience). The iT reg -cell differentiation conditions included 5 ng ml −1 rmTGF-β1 (R&D Systems) and 10 ng ml −1 rmIL-2 (R&D Systems). Flow cytometry Cytokines, transcriptional factors and surface markers were evaluated by flow cytometry with a FACSCanto II (BD Biosciences). To detect intracellular expression of IL-17A, IFN-γ in CD4 + T cells, lymph nodes or CNS (purified with Percoll) were first treated with 750 ng ml −1 ionomycin (Sigma), 50 ng ml −1 phorbol 12-myristate 13-acetate (PMA) (Sigma) and GolgiPlug (BD Biosciences) for 4–6 h at 37 °C. Cells were fixed and permeabilized with the Foxp3 Staining Buffer Set (eBioscience) or BD Cytofix/Cytoperm (BD Biosciences) and were stained with fluorescent antibodies. After washing, stained cells were assayed with a BD Biosciences FACSCanto II flow cytometer and data were analysed with FlowJo software. For flow cytometry, monoclonal antibodies against CD4 (clone GK1.5), CD8 (clone 53-6.7), CD62L (clone MEL-14), CD44 (clone IM7), CD25 (clone PC61.5), IL-17A (clone eBio17B7), IFN-γ (clone XMG1.2), Helios (22F6, Biolegend) and FoxP3 (clone FJK-16s) were from eBioscience and CD3 (clone 145-2C11) was from Biolegend. RNA reverse transcription and real-time quantitative PCR Total RNA was isolated using Trizol (Invitrogen) according to the manufacturer’s instructions. RNA was quantified spectrophotometrically, and 1 μg of total RNA was reverse transcribed into cDNA using SuperScript III (Invitrogen, Carlsbad, CA) in the presence of random hexamers and oligo dT primers (Invitrogen). The cDNA samples were distributed on plates at 200 ng per well and run in triplicate. qPCR was carried out with the FastStart Universal SYBR Green Master (Roche) in a ABI 7500 Fast Real-Time PCR system or ViiA 7 Real-Time PCR System (Applied Biosystems). Primer sequences were listed in Supplementary Table 1 . To measure mature miR-31 levels, 50 ng of total RNA was reverse-transcribed using the TaqMan miRNA reverse transcription kit, miR-31 RT primers and U6 snRNA (Applied Biosystems). The cDNAs were then analysed by qPCR using the TaqMan probes for miR-31 and U6 snRNA (Applied Biosystems). Quantification of relative miRNA expression was measured by the comparative CT (critical threshold) method, normalized to endogenous U6 expression and determined by the formula 2 −ΔΔCT . Chromatin immunoprecipitation assay ChIP assays were performed using the SimpleChIP enzymatic chromatin immunoprecipitation kit (Cell Signaling Technology) according to the manufacturer’s protocol with minor modifications. In brief, the cells were collected and crosslinked with 1% (v/v) formaldehyde for 10 min at room temperature. Subsequently, nuclei were isolated by the lysis of cytoplasmic fraction and chromatin was digested into fragments of 150–900 bp by micrococcal nuclease (400 gel units) for 20 min at 37 °C, followed by ultrasonic disruption of the nuclear membrane using a standard microtip and a Branson W250D Sonifier (four pulses, 60% amplitude, duty cycle 40%). The sonicated nuclear fractions were divided for input control and for overnight incubated at 4 °C with 5 μg either anti-FoxP3 Ab (FJK-16 s; eBioscience) or the negative control IgG (Cell Signaling Technology). After incubation with 30 μl of ChIP grade protein G-agarose beads for 2 h at 4 °C, the antibody-protein–DNA complexes were then eluted from the beads and digested by Proteinase K (40 μg) for 2 h at 65 °C, followed by spin column-based purification of the DNA. Finally, genomic DNA recovered from the ChIP assays were qPCR amplified with primers specific to the FoxP3-binding elements of the miR-31 promoter region. The primers used for detection of miR-31 promoter sequences were listed ( Supplementary Table 1 ). The specificity of each primer set was verified by analysing the dissociation curve of each gene-specific PCR product. In vitro T reg -cell suppression assay T reg cells were isolated from the spleen of mice by sorting with flow cytometry based on cell surface markers (CD4, CD25 and FoxP3 gfp ). Naive CD4 + T cells were isolated from the spleen of mice by sorting with flow cytometry based on cell surface markers (CD4 + , CD25 − , CD62L hi and FoxP3 gfp ). Splenocytes from RAG2 −/− mice lacking mature T and B lymphocytes were used as antigen presenting cells. The purified naive CD4 + T cells were labelled for 15 min at 37 °C with 10 μM CTV (Life Technologies) and the CTV-labelled T cells (1 × 10 5 ) were cultured in 96-well plates for 72 h together with an increasing ratio of sorted T reg cells in the presence of anti-CD3 (1 μg ml −1 ) plus γ-irradiated antigen-presenting cells (1 × 10 5 ). The suppressive function of T reg cells was determined by measurement of the proliferation of activated CD4 + effector T cells on the basis of CTV dilution. Generation of bone marrow chimeric mice Bone marrow cells were flushed from miR-31 fl/fl or cKO donor mice, and 5 × 10 6 T-cell-depleted bone marrow cells were transplanted into each C57BL/6J host mouse with total-body irradiation of 950 cGy in two divided doses. Chimeric mice reconstituted with bone marrow cells derived from either miR-31 fl/fl or cKO were subjected for EAE induction 8 weeks after the transplantation. Histology Spinal cords from miR-31 fl/fl or cKO EAE mice were fixed in 4% paraformaldehyde and paraffin embedded. Paraffin-embedded 5-μm sections of spinal cord were stained with haematoxylin and eosin or Luxol fast blue and then examined by light microscopy (Axio scope A1, Zeiss). Luciferase reporter plasmid The Gprc5a 3′-UTR was amplified using primers Gprc5a Forward, 5′- AATCTCGAGCTGTTGGGAAGAGTGGGAC -3′, Reverse, 5′- TCGGCGGCCGCAATAGTTGTGACCACATCTTTATTG -3′. The Gprc5a 3′-UTR genomic fragment was digested with XhoI-NotI and inserted into the corresponding sites of the psiCheck-2 Synthetic firefly luciferase reporter plasmid (Promega). This construct was also used to generate a miR-31 ‘seed’ mutant plasmid. The mutagenic primers used for Gprc5a were Mutant Forward, 5′- AATCTCGAGCTGTTGGGAAGAGTGGGAC -3′, Mutant Reverse, 5′- CAGCCCCACCGTTCTCGGCGGTG -3′. The correctness of all the plasmids was confirmed by sequencing. Luciferase assays All 3′ UTR reporter vectors were prepared by amplifying the 3′ UTRs of Gprc5a, followed by insertion into the psiCHECK-2 vector (Promega). Site-specific mutants were generated by PCR in the psiCHECK-2 vector (Promega). NIH3T3 cells were maintained in DMEM (HyClone) supplemented with 10% fetal bovine serum (HyClone), 2 mM glutamine, 100 IU ml −1 penicillin, 0.1 mg ml −1 streptomycin. NIH3T3 cells were seeded in the 24-well plates (1 × 10 5 cells per well) one day before transfection and then each well was transfected with a mixture of 100 ng 3′-UTR luciferase reporter vector and 50 pmol miRNA mimics or controls. Twenty four hours post transfection, the cells were lysed. Then, luciferase activity was measured using the Dual-Luciferase Reporter Assay System (Promega), using a Lumat 3 LB 9508 Single Tube Luminometer instrument (Berthold Technologies). Each experiment was performed in triplicate. The ratio of Renilla luciferase to Firefly luciferase was calculated for each well. Western blotting Cultured T cells and the CNS of mice were lysed in radio immunoprecipitation assay buffer supplemented with protease and phosphatase inhibitor cocktail (Thermo Scientific). Mouse anti-actin Ab (1:3,000) (Cell Signaling Technology), rabbit anti-Gprc5a Ab (1:1,000) (Dr Jiong Deng provided) were used. The signal was detected with Pierce ECL Western Blotting Substrate (Thermo Scientific) and GE ImageQuant LAS 4000 (GE Healthcare). Images have been cropped for presentation. Full size images are presented in Supplementary Fig. 8 . MicroRNA microarray analysis Naive T cells from 3 miR-31 fl/fl mice and 3 miR-31 fl/fl CD4 Cre mice were used to induce iT reg in vitro . Total RNA was isolated using RNeasy MiniKit (Qiagen). Mouse genome-wide cDNA microarray analysis was performed by Shanghai Biotechnology (Shanghai). Statistical analysis The data were analysed with GraphPad Prism 5 and were presented as the mean±s.e.m. Student’s t -test was used when two conditions were compared, and analysis of variance with Bonferroni or Newman–Keuls correction was used for multiple comparisons. Probability values of <0.05 were considered significant; two-sided tests were performed. Accession codes : Microarray data have been deposited in the GEO database under accession code GSE61938 . How to cite this article: Zhang, L. et al . MicroRNA-31 negatively regulates peripherally derived regulatory T-cell generation by repressing retinoic acid-inducible protein 3. Nat. Commun. 6:7639 doi: 10.1038/ncomms8639 (2015).